Electrochemically driven regioselective C−H phosphorylation of group 8 metallocenes Metallocenes are privileged backbones for synthesis and catalysis. However, the direct dehydrogenative C−H functionalization of unsymmetric metallocenes suffers from reactivity and selectivity issues. Herein, we report an electrochemically driven regioselective C−H phosphorylation of group 8 metallocenes. Mechanistic investigations indicate this dehydrogenative cross coupling occurs through an electrophilic radical substitution of the metallocene with a phosphoryl radical, facilitated by the metallocene itself. This work not only offers an efficient and divergent synthesis of phosphorylated metallocenes, but also provides a guide to interpret the reactivity and regioselectivity for the C−H functionalization of unsymmetric metallocenes. Since its discovery in the early 1950s [1] , [2] , [3] , [4] , [5] , ferrocene and its metallocene derivatives have received widespread attention owing to their broad applications in physics [6] , polymer science [7] , and medicine [8] , [9] . With regard to organic synthesis and catalysis, metallocene-based phosphines have proven to be privileged ligands or catalysts (Fig. 1a ) [10] , [11] , [12] , [13] , [14] , [15] , [16] , [17] , [18] , [19] , [20] . Although there are well-established methods for the synthesis of simple and unsubstituted metallocenes, the construction of substituted metallocene derivatives remains a challenge. Two general approaches have been used for the synthesis of substituted metallocenes. The first strategy is the coordination of substituted cyclopentadienyl precursors with the corresponding metal complex (Fig. 1b ) [21] , [22] , [23] . While reliable, this approach usually requires the multi-step synthesis of substituted cyclopentadienyl precursors and stoichiometric amounts of strong bases. The second strategy involves the C−H functionalization of the metallocene. The latter exhibits a better step economy but relies on strong bases or preinstalled directing groups [24] , [25] , [26] , [27] , [28] , [29] , [30] , [31] , [32] , [33] , [34] , [35] , [36] , [37] , [38] . Therefore, it is of great importance to address the challenges in developing an efficient and concise protocol for the construction of substituted metallocenes. Fig. 1: Synthesis of metallocene phosphine ligands. a Representative metallocenes and their derivatives. b General strategies for synthesizing substituted metallocenes and their derivatives. c Regioselectivity challenges in the direct dehydrogenative functionalization of unsymmetric metallocenes. d This work: Electrochemically driven regioselective C−H phosphorylation of group 8 metallocenes. Full size image Compared with the biscyclopentadienyl complex, the direct C−H functionalization of indenyl metallocenes poses an additional challenge in regiocontrol. Bearing six similar sp 2 C−H bonds on indenyl moiety, the 4-substituted indenyl metallocene is a representative unsymmetric substrate for C−H functionalization (Fig. 1c ). Theoretically, six possible regioisomers would be expected to form. We propose to develop a system to control the regioselectivity through site-selective differentiation of the six similar sp 2 C−H bonds. Based on the principle of mass conservation, this direct C−H functionalization will generate one molar equivalent of hydrogen gas or an associated byproduct. Usually, an external oxidant is required as a hydrogen scavenger. Meanwhile, electrochemical synthesis [39] , [40] , [41] , [42] , [43] , [44] , [45] , [46] , [47] , [48] , [49] , [50] , [51] is a powerful method to facilitate oxidative cross-coupling reactions [52] , [53] , [54] , [55] , [56] , [57] , [58] under external-oxidant-free conditions through anodic oxidation. Specially, electrochemical phosphorylation [59] , [60] , [61] , [62] , [63] , [64] , [65] , [66] , [67] , [68] , [69] , [70] has emerged as a complementary approach to conventional methods for forming C−P bonds. Here, we report an efficient regioselective C−H phosphorylation of group 8 metallocenes (Fig. 1d ). This oxidative cross-coupling protocol features broad substrate scope and mild conditions while avoiding the use of directing groups and external oxidants. Reaction optimization Initially, under electrolysis conditions, benzoferrocene 1a and diphenyl phosphine oxide 2a were selected as model substrates to optimize the reaction. 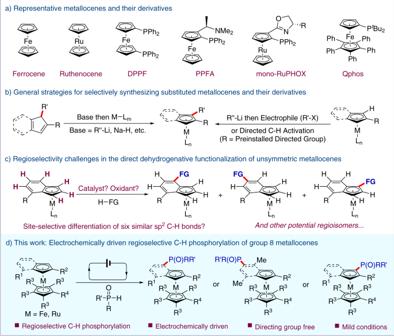Fig. 1: Synthesis of metallocene phosphine ligands. aRepresentative metallocenes and their derivatives.bGeneral strategies for synthesizing substituted metallocenes and their derivatives.cRegioselectivity challenges in the direct dehydrogenative functionalization of unsymmetric metallocenes.dThis work: Electrochemically driven regioselective C−H phosphorylation of group 8 metallocenes. The reaction was conducted under constant current in an undivided cell equipped with a reticulated vitreous carbon (RVC) anode and a platinum plate cathode (Table 1 ). Using n Bu 4 NOAc as the electrolyte, monophosphorylated product 3a was obtained in high regioselectivity and 73% yield in MeOH (entry 1). It is notable that small amounts of over phosphorylated products ( 4a , 5a , and 6a ) were obtained. No desired reaction occurred in the absence of current (entry 2). Other electrode materials, including Pt and graphite anode, were all found to be less effective in terms of reactivity (entries 3 and 4). The use of an alternative electrolyte, such as n Bu 4 NBF 4 , or LiClO 4 •3H 2 O lowered reaction efficiency (entries 5 and 6). Increasing the current to 3.0 or 5.0 mA had a negative effect on selectivities and favored the formation of bisphosphorylated products 4a – 6a (entries 7 and 8). On the other hand, conducting the electrolysis without Et 3 N resulted in a lower yield (entry 9). Other basic additives such as NaOAc and K 3 PO 4 failed to give better results (entries 10 and 11). Solvents such as TFE (Trifluoroethanol), DCE (1,2-Dichloroethane), and MeCN were screened as well, but lower yields were obtained (entries 12–14). Notably, the electrochemical reaction could also be performed at RT (room temperature), although with a slight decrease in yield (entry 15). And the use of stoichiometric oxidants (e.g., AgF, MnO 2 , and DDQ (1,2-Dichloro-4,5-Dicyanobenzoquinone), etc.) for this phosphorylation gave low yields (See Supplementary Table 1 in Supporting Information). Table 1 Optimization of reaction conditions a . Full size table Substrate scope Having identified optimized conditions, we next evaluated the phosphorylation of different benzoferrocenes with diphenyl phosphine oxide 2a (Fig. 2a ). The presence of a Br, Me, or Ph group at the α-position of the aryl ring of 1-methylbenzoferrocences were all well tolerated to afford the phosphorylated products in decent yields ( 3a – 3c ). It should be noted that even when either Cp (cyclopentadienyl) or phenyl rings on the benzoferrocene substrates were naked, the phosphorylation still occurred at the α -position of phenyl ring ( 3d – 3f ). Some of the relatively low yields ( 3d and 3e ) were due to low conversion or decomposition of substrates rather than regioselective issues. These results suggest that the Br atom on model substrate 1a does not act as an activating or directing group in this protocol. Due to its electron deficiency, the aza-benzoferrocene substrate was not applicable in this case ( 3g ). Fig. 2: Substrate scope. a Scope of benzoferrocenes for C4-phosphorylation. b Scope of phosphine oxides for C4-phosphorylation of benzoferrocenes. c Scope of phosphine oxides for C5-phosphorylation of benzoferrocenes. a Reaction with 2.5 mA, 6 h (2.8 F/mol). b Reaction with 3.0 mA, 10 h (5.6 F/mol). Brsm refers to the yield based on the recovered starting material. Full size image Subsequently, we turned our attention to the investigation of the scope of phosphine oxides with Br-substituted benzoferrocenes, which was good for further derivatization. As shown in Fig. 2b , phosphine oxides containing electron-donating or electron-withdrawing groups, such as -Me, - t Bu, -Ph, -OCF 3 , -Cl, and -F, at the para position of the aryl components, all resulted in good yields ( 3h – 3m ). Likewise, substrates with substituents at the meta-position of the aryl components also exhibited good reactivities and delivered the corresponding products in 60–75% yields ( 3n – 3q ). Delightfully, the reaction also demonstrated good tolerance for the phosphine oxide bearing a heterocyclic 2-thiophenyl group ( 3r ) which is usually problematic under transition metal catalysis. To our surprise, the desired reactions also worked when benzoferrocenes with the α -positions of the aryl components blocked were subjected to the standard conditions (Fig. 2c , 3s – 3w ). Less than 10% of the corresponding 2-phosphorylated products could be observed for these substrates. Meanwhile, over phosphorylations and decomposition of substrates resulted in the relatively low yields ( 3s – 3w ). The regioselectivity and molecular structures of 3q and 3v ′ were unambiguously determined by single-crystal X-ray diffraction analysis. Additionally, the current electrochemical protocol was also suitable for the phosphorylation of simple ferrocene substrates (Fig. 3a ). Substrates bearing either electron-donating or electron-withdrawing groups at the phenyl rings of phosphine oxides were all tolerated and gave the phosphorylated products in 48–75% yields ( 8a – 8g ). 1-Naphylphosphine oxide was applicable to the standard condition as well ( 8h ), while subjecting 2-thiophenyl phosphine oxides to the reaction could only deliver the desired product in a 38% yield ( 8i ). For the substrate 1,1’-dibenzylferrocene, the products of o -phosphorylation and m -phosphorylation were isolated respectively in 1:2.8 ratio. Next, pentamethylferrocene and their analogs were tested with various phosphine oxides (Fig. 3b ). These reactions proceeded successfully and all occurred at the bare Cp rings, leading to products in 36–74% yields ( 8k – 8y ). Unfortunately, the phosphorylation of ruthenocene initially failed due to its low solubility in MeOH. To overcome this drawback, DCE was chosen as solvent and LiClO 4 •3H 2 O was selected as an electrolyte in this case. Under the modified condition, ruthenocene reacted with a series of phosphine oxides smoothly and delivered products in decent yields ( 10a–10g ), which further highlights the generality of the current strategy. The structure of ruthenocenyl phosphine oxide 10e was also further confirmed by single-crystal X-ray diffraction analysis. Fig. 3: Substrate scope for C−H phosphorylation of ferrocenes and ruthenocenes. a C−H phosphorylation of ferrocenes (Condition A). b C−H phosphorylation of pentasubstituted ferrocenes (Condition A). c C−H phosphorylation of ruthenocenes (Condition B). a Reaction with 2.0 mA, 12 h (4.5 F/mol). b Reaction with 2.5 mA, 12 h (5.6 F/mol). c Reaction with 4.0 mA, 12 h (9.0 F/mol). d Regioselectivity o : m = 1:2.8. e Reaction with 6.0 mA, 10 h (11.2 F/mol). Full size image Mechanistic investigations To probe the mechanism of this electrochemically enabled C−H phosphorylation of metallocenes, preliminary mechanistic investigations have been conducted (Fig. 4 ). The addition of radical scavengers TEMPO (2,2,6,6-tetramethylpiperidinoxy) to the reaction mixture almost suppressed the reactivity (Fig. 4a , entry 2 vs 1). Using BHT (butylated hydroxytoluene) and 1,2-diphenylethylene as a radical scavenger, the phosphorylated products 12a and 12b were isolated in 25 and 18% yield respectively (entries 3–4) [71] . Besides, radical clock reaction with 2 equiv. of (1-cyclopropylvinyl)benzene ( 11c ) led to the ring-opened product 12c (entry 5) [72] . The above experiments are strongly suggestive of a phosphinyl radical species being involved in this reaction. Fig. 4: Mechanistic investigations. a Radical inhibition and capture experiments. b Control experiments of ferrocenium. c Kinetic studies. d Catalytic C−H phosphorylation of naphthalene facilitated by ferrocene. e Cyclic voltammograms (CVs). Full size image In order to get insight into this electrochemical process, control experiments of ferrocenium were carried out (Fig. 4b ). Conducting electrolysis by replacing ferrocene with ferrocenium 13a under the standard conditions gave a 50% yield of 8a accompanied by 7a (entry 1). Notably, an 18% yield of 8a could be obtained without electricity. A similar phenomenon was also observed in the control experiments with 7d (entries 3–4). Interestingly, some amount of phosphorylation product 8r was still obtained in the absence of electricity. These results suggest that this phosphorylation may undergo through the ferrocenium species. Kinetic studies on the coupling of 7a with 2a showed phosphorylation product 8a was generated continuously at the first 4h (Fig. 4c ). Surprisingly, a small amount of 16 was observed when the kinetic studies of phosphorylation of 7a were performed using naphthalene as the internal standard (Fig. 4 c, d ). Only 2% phosphorylated naphthalene could be obtained without 7a under standard conditions (Fig. 4d , entry 1). The addition of a catalytic amount of ferrocene 7a or ferrocenium 13a helped the formation of 16 (entries 2 and 3). Through rough optimization with ferrocene as a redox catalyst, the yield of 16 was improved to 54% (entries 4 and 5). Therefore, the above experiments suggested that the ferrocene could act as a redox catalyst in phosphorylation. Next, cyclic voltammograms (CVs) of 7a were conducted under different conditions to gain mechanistic insight (Fig. 4e ). The oxidation potential of ferrocene 7a was 0.44 V (curve I). Although compound 2a exhibited no apparent peak from 0 to 1.6 V (Supplementary Fig. 1 , curve V, Supporting Information) [50] , [63] , [69] , 2a showed an oxidative potential at 1.25 V in the presence of the base NaOMe (Supplementary Fig. 1 , curve VI, Supporting Information). No significant change on the CVs of 7a was observed in the presence of 2a (curve II) and adding Et 3 N had also no remarkable change (curve III). However, a catalytic current could be observed when 7a was mixed with 2a and NaOMe (curve IV) [39] . A comparison of curves IV and VI (Fig. 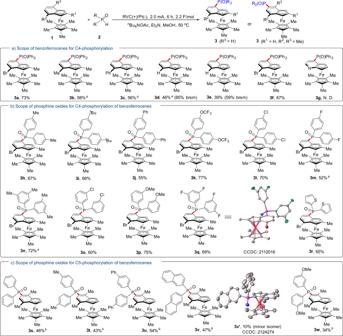Fig. 2: Substrate scope. aScope of benzoferrocenes for C4-phosphorylation.bScope of phosphine oxides for C4-phosphorylation of benzoferrocenes.cScope of phosphine oxides for C5-phosphorylation of benzoferrocenes.aReaction with 2.5 mA, 6 h (2.8 F/mol).bReaction with 3.0 mA, 10 h (5.6 F/mol). Brsm refers to the yield based on the recovered starting material. S1 ), the voltammogram of the conjugate base of 2a , suggested that the current increase of curve IV did not result from the oxidation of phosphine oxide anion. The above results suggest that the addition of NaOMe facilitates the oxidation of 2a with ferrocenium. Notably, MeO − is assumed to be generated at the cathode through the reduction of MeOH. Based on the CVs of the metallocene substrates and products, the observed oxidation potentials could account for the reactivity difference between electron-rich and electron-deficient metallocenes (Fig. 4e ). Based on the experimental results above and literature precedent, a proposed mechanism is shown in Fig. 5 . The electrolytic process begins with the anodic oxidation of 7a that produces ferrocenium ion B . Meanwhile, the addition of Et 3 N facilitates deprotonation of 2 for the formation of anion A . A first single-electron transfer (SET) between anion A and ferrocenium ion B generates phosphinyl radical C and ferrocene 7a . Subsequently, the in situ formed phosphinyl radical C adds to ferrocene 7a to yield radical species D . A second SET between radical D and ferrocenium ion B delivers the desired phosphorylation product 8 and regenerates ferrocene 7a for the next cycle. The hydrogen is released at the cathode. Therefore, an external oxidant is not required in this cross dehydrogenative phosphorylation. Fig. 5: Proposed mechanism. a Proposed mechanism. b Regioselectivity interpretation. Full size image In order to interpret the unexpected high regioselectivity in the phosphorylation of benzoferrocenes 1 , the structural properties of 1e and 1h have been shown in Fig. 5b . Some important bond lengths are given according to the single-crystal X-ray diffraction analysis. For these substrates, the bond lengths of C(5)=C(6) and C(7)=C(8) are between 1.35–1.37 Å which are shorter than that of benzene (1.39 Å). The bond lengths for the rest of the C−C bonds on the indenyl motif are ~1.42 Å. These results suggest higher electron density is located around C(5)=C(6) and C(7)=C(8) and makes them more nucleophilic. Taking 1a as the example for regioselectivity interpretation, the four most likely radical species D ( D1–D4 of 1a ) will be expected to form via the reaction of phosphinyl radical C with benzoferrocene 1a . Based on the distribution of electron density on the indenyl motif, D1-1a is the least favored species to generate. Owing to the steric hindrance of the bromine atom, the formation of D4-1a is not preferred. Stronger ability on the stabling the allylic radical species make D2-1a preferentially yielded over D3-1a . The electron density distribution on the indenyl motif also results in the formation of 6a as the major bisphosphorylated side product. Finally, gram-scale preparations of 8a (1.02 g) and 3a (1.74 g) were carried out to demonstrate the efficacy of this protocol (Fig. 6 a, b ). Further synthetic elaborations of these materials were conducted to show the synthetic utility. For instance, a strong single-electron oxidant 17 could be synthesized through the oxidation of 8a with BQ (1,4-Benzoquinone) in the presence of HPF 6 [73] . Meanwhile, ferrocene-based phosphine 18 could be prepared via reduction of 8a with HSiCl 3 . Through a selective sp 2 C−H activation, amination product 19 was produced under Ir catalysis [74] . Besides, 1,1′-disubstituted ferrocenyl phosphine oxide 20 could be obtained with high regioselectivity through Friedel–Crafts acylation of 8a . Further reduction of 20 with LiAlH 4 delivered alcohol 21 . For the reduction of 3a , phosphine product 22 was isolated with a bromine atom intact. Additionally, 3b could be obtained via Ni-catalyzed Kumuda coupling reaction. Interestingly, with n Bu 4 NPF 6 as the electrolyte, a selective sp 3 C−H etherification of 3a occurred efficiently in MeOH to deliver product 23 [75] . Furthermore, another different phosphinyl moiety can be installed on benzoferrocenes to obtain highly functionalized 24 , which would otherwise be challenging to synthesize via traditional means. Fig. 6: Scale-up preparations and synthetic transformations. a Scale-up preparation and synthetic transformation of 8a . b Scale-up preparation and synthetic transformation of 3a . Full size image In this work, we have developed an electrochemically driven regioselective cross-coupling of group 8 metallocenes with phosphine oxides. Without preinstalled directing groups or pyrophoric alkyl lithium reagent, over 60 examples of phosphorylated (benzo)ferrocenes and ruthenocene are easily accessed through this intermolecular dehydrogenative C−H phosphorylation. Mechanistic studies suggest that the desired C−P bond is constructed through a radical substitution between phosphoryl radical and metallocene. Meanwhile, the metallocene acts as a single-electron transfer reagent for radical generation and quenching. The high regioselectivity for the C−H phosphorylation of benzoferrocenes is a consequence of the unequal electron density distribution on the indenyl motif. General procedures for electrochemically driven C−H phosphorylation ferrocenes or benzoferrocences (Method A): In an oven-dried undivided three-necked flask equipped with a stir bar, ferrocenes or benzoferrocenes (0.20 mmol), diphenyl phosphine oxide (0.40 mmol), Et 3 N (0.40 mmol), n Bu 4 NOAc (0.20 mmol), and MeOH (4 mL) were combined. The flask was equipped with RVC (100 PPI, 15 mm × 10 mm × 5 mm) as the anode and platinum plate (10 mm × 10 mm × 0.3 mm) as the cathode under an inert atmosphere in a nitrogen glove box. The flask was capped with a septum. The reaction mixture was stirred and electrolyzed at a constant current of 2.0–4.0 mA at 50 o C for 6–12 h. Upon reaction completion, the reaction crude was washed with water and the product was extracted with dichloromethane (10 × 3 mL). The organic layers were combined, dried over Na 2 SO 4 , and concentrated. The pure product was obtained after flash column chromatography on silica gel (petroleum: ethyl acetate = 1:1–4:1). General procedures for electrochemically driven C−H phosphorylation ruthenocene (Method B): In an oven-dried undivided three-necked flask equipped with a stir bar, ruthenocenes (0.20 mmol), diphenyl phosphine oxide (0.40 mmol), Et 3 N (0.40 mmol), LiClO 4 •3H 2 O (0.30 mmol), and DCE (4 mL) were combined. The flask was also equipped with RVC (100 PPI, 15 mm × 10 mm × 5 mm) as the anode and platinum plate (10 mm × 10 mm × 0.3 mm) as the cathode under inert atmosphere in a nitrogen glove box. The flask was capped with a septum. The reaction mixture was stirred and electrolyzed at a constant current of 6.0 mA at 50 o C for 10 h. Upon reaction completion, the reaction crude was washed with water and the product was extracted with dichloromethane (10 mL × 3). 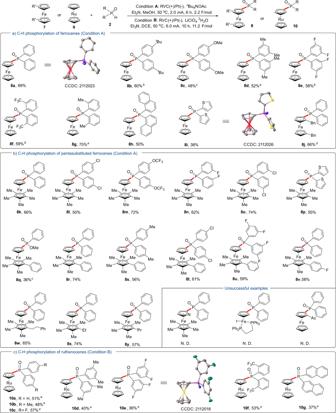Fig. 3: Substrate scope for C−H phosphorylation of ferrocenes and ruthenocenes. aC−H phosphorylation of ferrocenes (Condition A).bC−H phosphorylation of pentasubstituted ferrocenes (Condition A).cC−H phosphorylation of ruthenocenes (Condition B).aReaction with 2.0 mA, 12 h (4.5 F/mol).bReaction with 2.5 mA, 12 h (5.6 F/mol).cReaction with 4.0 mA, 12 h (9.0 F/mol).dRegioselectivityo:m= 1:2.8.eReaction with 6.0 mA, 10 h (11.2 F/mol). 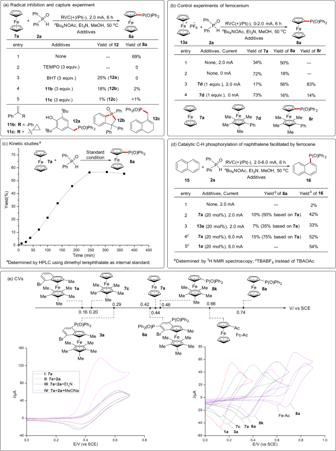Fig. 4: Mechanistic investigations. aRadical inhibition and capture experiments.bControl experiments of ferrocenium.cKinetic studies.dCatalytic C−H phosphorylation of naphthalene facilitated by ferrocene.eCyclic voltammograms (CVs). The organic layers were combined, dried over Na 2 SO 4 , and concentrated. 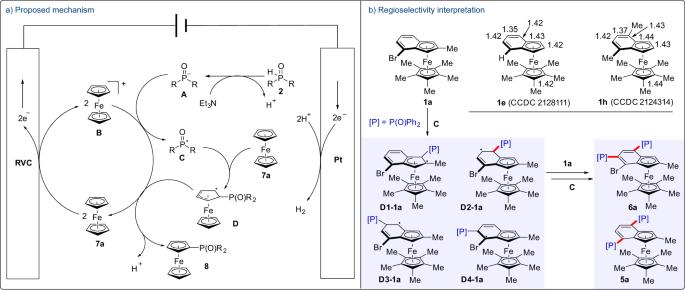Fig. 5: Proposed mechanism. aProposed mechanism.bRegioselectivity interpretation. 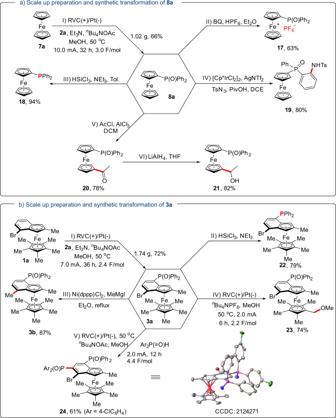Fig. 6: Scale-up preparations and synthetic transformations. aScale-up preparation and synthetic transformation of8a.bScale-up preparation and synthetic transformation of3a. The pure product was obtained after flash column chromatography on silica gel (petroleum: ethyl acetate = 1:1).